Substrate stiffness-modulated registry phase correlations in cardiomyocytes map structural order to coherent beating Recent experiments show that both striation, an indication of the structural registry in muscle fibres, as well as the contractile strains produced by beating cardiac muscle cells can be optimized by substrate stiffness. Here we show theoretically how the substrate rigidity dependence of the registry data can be mapped onto that of the strain measurements. We express the elasticity-mediated structural registry as a phase-order parameter using a statistical physics approach that takes the noise and disorder inherent in biological systems into account. By assuming that structurally registered myofibrils also tend to beat in phase, we explain the observed dependence of both striation and strain measurements of cardiomyocytes on substrate stiffness in a unified manner. The agreement of our ideas with experiment suggests that the correlated beating of heart cells may be limited by the structural order of the myofibrils, which in turn is regulated by their elastic environment. The mechanical microenvironment of a cell influences key aspects of cell functionality and structure [1] , [2] , [3] . In particular, both the morphology and beating of embryonic heart muscle cells or cardiomyocytes have been observed to depend sensitively on the rigidity of the substrate on which they are cultured [4] , [5] , [6] , [7] , [8] . Muscle fibres consist of oriented myofibrils, periodic arrays of sarcomeres, which are the contractile units of muscle, and consist of interdigitated thick and thin filaments made of myosin and actin, respectively [9] (see Fig. 1 ). Like other striated muscle tissue, cardiomyocytes contain fibrils that are not only oriented (actomyosin stress fibres in other tissue types, such as fibroblasts, can also be ‘nematically oriented’ in this sense) and periodic along their length, but are also registered across neighbouring fibrils in a manner that is analogous to ‘smectic order’ in liquid crystals, and as such, are an example of highly ordered active matter in biology. This registry is manifested by alignment across different fibrils of the location of their z-discs, molecular assemblies that cross-link the actin filaments, which gives cardiac muscle tissue its characteristic striated appearance. We describe this registry quantitatively as a phase-order parameter and show that it has implications for the correlated beating of a cardiomyocyte. Understanding the mechanical influences on myofibrilligenesis, the process by which myofibrils form and organize into such a well-ordered structure in muscle tissue, and its implications for the contractile function of cardiomyocytes, is an extremely important problem in cardiac physiology, regenerative medicine [10] and developmental biology [11] . 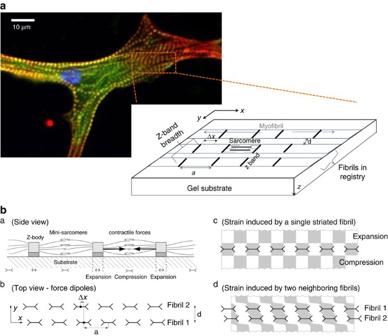Figure 1: Experimental setup and conceptual sketch of muscle cell on a gel substrate. (a) E7 chick cardiomyocyte cultured on collagen-I-coated 11 kPa polyacrylamide gel and stained for sarcomeric alpha actinin (green), filamentous actin (red) and DNA (blue) to visualize myofibril striations. The ‘blow-up’ shows a schematic illustration of the experimental setup. Here, three aligned, parallel myofibrils are shown; the two fibrils indicated are in registry, whereas the third is off registry by a distance Δx. Each fibril is made of a repeating sarcomere unit (comprising alternating actin and myosin filaments, here shown as dashed and solid lines, respectively). The distance between neighbouring z-discs along a fibril, that is, the unit cell size or length of a sarcomere is denoted asa, whereasdis the transverse inter-fibril distance. (b) Illustration of the same from 2D perspectives. Figure (b) is reproduced with permission from ref.18. Figure 1: Experimental setup and conceptual sketch of muscle cell on a gel substrate. ( a ) E7 chick cardiomyocyte cultured on collagen-I-coated 11 kPa polyacrylamide gel and stained for sarcomeric alpha actinin (green), filamentous actin (red) and DNA (blue) to visualize myofibril striations. The ‘blow-up’ shows a schematic illustration of the experimental setup. Here, three aligned, parallel myofibrils are shown; the two fibrils indicated are in registry, whereas the third is off registry by a distance Δ x . Each fibril is made of a repeating sarcomere unit (comprising alternating actin and myosin filaments, here shown as dashed and solid lines, respectively). The distance between neighbouring z-discs along a fibril, that is, the unit cell size or length of a sarcomere is denoted as a , whereas d is the transverse inter-fibril distance. ( b ) Illustration of the same from 2D perspectives. Figure ( b ) is reproduced with permission from ref. 18 . Full size image The development of individual myofibrils as oriented, periodic structures is a complex process [11] , [12] , [13] , [14] involving a host of mechanisms, including biochemical factors as well as active, contractile stress generation and mechanical coupling to the extracellular matrix [15] . Experiments by Engler et al . [16] suggest that the secondary organization or registry of neighbouring myofibrils is a mechanically regulated process, as the maximum number of well-striated muscle cells in culture occurs on an optimally rigid substrate (which is neither too soft nor too rigid). The observation of strong striations indicates the local registry of fibrils. Recent measurements by Majkut et al . [8] of both registry correlations of neighbouring myofibrils and the substrate deformation induced by a contracted cardiomyocyte in culture during beating show that the striations and the strain are each maximal at particular (but different) values of the substrate elasticity E . Similar correlated changes in registry and contractility have also been anecdotally noted by Hersch et al . [17] for rounded myocytes on soft substrates and seen by directly varying cell shape [18] . In addition, Majkut et al . [8] observe that the curves for the striations as a function of the substrate rigidity are narrower for less ordered (earlier time) situations such as premyofibrils compared with more developed myofibrils. We explain these trends in the peak width by including the disordering effect of noise (as well as orientational disorder) in a model for the interaction between fibrils that is mediated by the deformations that they induce in the substrate [19] . More importantly, our model maps the observed values of the registry striations to that of the measured beating strain as functions of the substrate rigidity, and thus reconciles two sets of data that are apparently very different. The success of our theoretical ideas in reconciling the two independent measurements of striation and contractile strain suggests that the correlated beating of a heart cell may be related to the registry of its myofibrils, which in turn is regulated by their elastic environment. Muscle registry in noisy environments The tendency of neighbouring myofibrils to register can be understood theoretically in terms of mechanical forces exerted on a sarcomere by nearby, contractile, muscle fibrils via elastic deformations of the substrate. Each muscle fibril can be considered as a periodic array of active, contractile, force dipoles. The theoretical construct of an active force dipole [20] provides a coarse-grained model for a cell’s cytoskeletal contractility, and has been applied to understand the mechanical response of single cells in various situations [21] , such as its orientation under an external stretch [22] , or the dependence of the polarization (nematic order) of its stress fibres on substrate rigidity [23] that deforms the elastic substrate via acto-myosin contractile forces exerted at the adhesion sites of the z-discs [19] . The transduction of this force induces a periodic strain field in the substrate with alternating regions of compression and expansion (see Fig. 1b ). The adhesions that connect the z-discs of the sarcomeres to the substrate are acted upon by forces from the substrate that arise from the deformations induced by the contractility of the neighbouring fibre. This effect can also be thought of in terms of the elastic energy of the adhesions in the stress field caused by the neighbouring fibre. This energy when a neighbouring parallel myofibril is out of registry by a distance Δ x is given by (see ref. 19 for detailed derivation), Here a is the periodicity of the force dipole density of the fibril(typically 2 μm for mature myofibrils)and κ =4 η /(1+ η ) 2 is a mechanical parameter defined in terms of η = E / E *, the elasticity of the substrate normalized by the substrate rigidity E * at which the force generated by a contractile unit saturates. Measurements [24] and models [22] of the dependence of the force generated by cells on elastic substrates suggest that one can write the force dipole density as a function of rigidity as: ρ ( E )= ρ */(1+ E */ E ), where ρ * is the saturated force dipole density (1 D ) of a fully contractile cell (as defined here, the force dipole density per unit length, ρ has units of force). This relation is responsible for the dependence of the interaction energy on substrate elasticity, as expressed in equation (1), where U int is the energy scale of the elastically mediated, force dipole interactions, given by, . Here Φ is a transverse strain propagation factor that is positive and of order unity for typical values of the Poisson’s ratio but does not depend on E . However, Φ does depend on the spacing between adjacent fibres [19] . Although the calculations here are performed assuming parallel fibres (as in Fig. 1 ), the lack of orientational (nematic) order that is observed in experimental systems can be taken into account to first order, by averaging Φ over the range of distances present in two fibres that are locally parallel but globally disordered with respect to their orientation and hence spacing. Nematic disorder in the system would then be reflected by a smaller value of Φ and hence of the interaction strength. Equation (1) suggests that perfect registry between fibrils, Δ θ =2 π Δ x / a , is mechanically the most favourable state. Although stochastic forces arising from actin polymerization or myosin contractility could move a sarcomere in a random direction, the elastic force would tend to drive it in a direction that lowers the mechanical work it is required to perform. If, for example, a sarcomere were in a region where it would require more work to maintain its contractility, a stochastic deviation from that position (due to active noise in the system) could result in elastic forces that bring it closer to registry, where the work required to deform the substrate in the presence of the neighbouring sarcomeres is smaller. The elastic forces are then expected (in the absence of noise) to drive the sarcomere into perfect registry with the neighbouring fibril, even for very small values of the elastic interaction strength. Although the forces exerted on a sarcomere by a neighbouring, periodic assembly of similar sarcomeres, modelled as a line of force dipoles, on an elastic substrate tend to register them, the forces produced by both thermal noise and molecular motors such as myosin are inherently stochastic in nature [25] , and introduce local fluctuations that tend to counteract the tendency to register. At long time scales, where both the thermal and ‘active’ noise can be regarded as delta correlated, the overall noise can be quantified as an effective temperature [26] , [27] , [28] , [29] T N . The extent of registry of two neighbouring myofibrils can then be predicted from a statistically averaged registry ‘order parameter’, S =‹cos(2 π Δ x / a )›= S ( βκ ), with a noise parameter β = U int /( k B T N ) that results from the competition between the elastic interactions given by equation (1) and the effective noise temperature, and κ is a peaked function of the substrate elasticity as defined earlier. For perfect registry between a pair of fibrils, such as when there is no noise, the order parameter S =1, while it is expected to go to zero when the effective temperature is much higher than the elastic interaction energy. The parameter β reflects not only the strength of the elastic interactions but also the extent of nematic order of neighbouring fibrils as explained above. The mechanical parameter η defined earlier is responsible for the peak in S versus E , and the effective Boltzmann factor β decides its width. The z-band breadth (zbb), as defined in ref. 8 , is a key experimentally observable metric of myofibril registry corresponding to statistical correlations of registry across neighbouring fibrils, and is closely related to the theoretical order parameter S defined above. When neighbouring fibrils are in perfect registry with each other, that is, for the fully ordered situation with S =1, their z-discs line up and appear as one indistinguishable stripe within the resolution of the imaging technique employed, as illustrated in Fig. 1a . The zbb in this case would correspond to the total thickness of two neighbouring myofibrils denoted by w 2 , which includes the spacing between them which is about 200–400 nm. In the situation where fibrils are not registered at all, that is, for S =0, the zbb would just correspond to the thickness of the z-disc of a single myofibril w 1 , which is about 1 μm. Adjusting for this offset and using a value of w 2 =2.3 μm for the total zbb of two perfectly registered fibrils, we use a linear interpolation zbb=( w 2 – w 1 ) S + w 1 , to obtain the values of the order parameter S (plotted in Fig. 2 ) from the corresponding experimentally observed zbb value in Ref. 8 [8] . 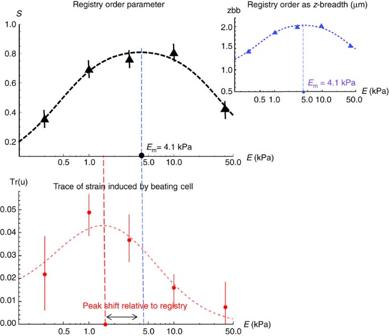Figure 2: Experimental observations of striation and matrix strain for a beating cardiomyocyte versus substrate elasticity. The upper panel shows the theoretical registry order parameter valuesScalculated from the z-band breadth measurement(zbb) data (shown as an inset of the upper panel with blue triangles) reported inFig. 4fof ref.8as solid, black, triangles at different values of substrate elasticity. The dashed line is an interpolated guide to the eye that connects the data points to within the error bars and determines the peak position to be at a substrate elasticity value ofEm=4.1±0.2 kPa, whereas the half maximum is reached at 0.4 and 50 kPa. TheSvalues are calculated from the zbb values using the fact that the theoretical minimum and maximum zbb values correspond to the breadth of a single myofibril (1 μm) and the combined breadth of two myofibrils (2.3 μm) in the totally disordered and fully registered cases, respectively. The measured average strain in the substrate around the cell is plotted as solid red dots with the corresponding error bars (lower panel). The strain values show a peak at a substrate elasticity of around 1.4 kPa and reach half maximum at 0.2 and 8 kPa. Together, these data sets demonstrate that both strain and registry depend on substrate elasticity and, respectively, show peaks atdifferentvalues of the substrate rigidity, but the exact nature of the dependence of strain on substrate rigidity is different from that of registry (showing very different widths at half maxima values for example). Figure 2: Experimental observations of striation and matrix strain for a beating cardiomyocyte versus substrate elasticity. The upper panel shows the theoretical registry order parameter values S calculated from the z-band breadth measurement(zbb) data (shown as an inset of the upper panel with blue triangles) reported in Fig. 4f of ref. 8 as solid, black, triangles at different values of substrate elasticity. The dashed line is an interpolated guide to the eye that connects the data points to within the error bars and determines the peak position to be at a substrate elasticity value of E m =4.1±0.2 kPa, whereas the half maximum is reached at 0.4 and 50 kPa. The S values are calculated from the zbb values using the fact that the theoretical minimum and maximum zbb values correspond to the breadth of a single myofibril (1 μm) and the combined breadth of two myofibrils (2.3 μm) in the totally disordered and fully registered cases, respectively. The measured average strain in the substrate around the cell is plotted as solid red dots with the corresponding error bars (lower panel). The strain values show a peak at a substrate elasticity of around 1.4 kPa and reach half maximum at 0.2 and 8 kPa. Together, these data sets demonstrate that both strain and registry depend on substrate elasticity and, respectively, show peaks at different values of the substrate rigidity, but the exact nature of the dependence of strain on substrate rigidity is different from that of registry (showing very different widths at half maxima values for example). Full size image Fitting the experimentally measured registry order and strain values separately to the corresponding theoretical expressions for S ( βκ ) and strain, respectively, would require us to have the noise β as a fitting parameter. However, as discussed later on, the more important point is that we can map the registry to the strain data without any need for fits and without specifying a value for β . Mapping structural registry to beating strain Majkut et al . [8] measured the deformations induced during the beating of cardiomyocytes (relative to the relaxed state) by imaging the displacements of a set of fiducial points on the periphery of the cell. The experimentally measured strains also show a peak when plotted versus the substrate elasticity but the peak occurs at a lower substrate elasticity value (around 1.5 kPa), whereas that of the registry striations occurs at E m =4 kPa. The position of the peak in registry corresponds in our theory to the substrate elasticity at which this particular type of cardiomyocytes (of embryonic chicks) become fully contractile, E *. The value of E *=4 kPa is comparable to the corresponding saturation rigidity of 10 kPa for cardiomyocytes in neonatal rats [5] . Figure 2 shows that besides differing in their peak positions, the shape and width of the registry and strain curves plotted versus substrate elasticity are significantly different, the width at half maximum being about 50 and 8 kPa, respectively. We now show how our model allows one to map the structural information (registry as a function of substrate elasticity) to cardiomyocyte function (beating strain as a function of the substrate rigidity), and thus reconcile the top and bottom panels of Fig. 2 . Assuming that only fibrils that are in registry beat synchronously, so that only registered fibrils produce strains that add coherently, we can predict the experimental measurements of beating strain versus substrate rigidity with the same noise and elastic parameters that characterize the structural data of Fig. 2 . In the Methods section, we show how the inclusion of noise via an effective Boltzmann distribution with the interaction of equation (1) predicts a registry correlation length ξ that is a measure of the number of fibres that are in mutual registry because of their elastically mediated interactions. As this depends on the competition of the elastic interactions and the noise, the correlation length ξ varies with the substrate rigidity. We expect ξ to be larger for more registered fibrils, and our statistical mechanics analogy (see Methods) shows that it can be related to the nearest-neighbour registry correlations S as ξ ( S )~− d /log( S ), where d is the spacing between neighbouring fibrils. More strongly correlated fibrils beat more coherently thus producing stronger strains in the substrate. This predicts that the strain should be an increasing function of ξ. Assuming that fibrils become uncorrelated and beat with random phases relative to each other beyond a distance of separation equal to the correlation length ξ, the average strain is proportional to , where N is the number of such independently beating groups of fibrils. This number N in turn is inversely related to the correlation length, N ~1/ ξ , because stronger correlations imply larger groups of fibres, which beat together and thus fewer independently beating groups. The trace of the strain field, Tr ( u )= u xx + u yy + u zz , where u ij is a component of the strain tensor, produced by the beating of such groups of fibrils can be mapped onto the structural registry characterized by the order parameter S through the relation (see Methods for the details of derivation): showing that the strain peak shifts relative to the striation peak because of the additional factor of 1/( E + E *), which originates from the fact that strain goes inversely as substrate elasticity E but the contractile forces saturate on stiff substrates as E /( E + E *). This contributes a factor of 1/ E for asymptotically large E that makes the strain peak narrower than the one in registry as shown in Fig. 2 . The dependence of strain on elasticity through the registry correlation length ξ is much weaker because of the logarithm function. An experimental measure of ξ is hard to obtain as correlations beyond the nearest-neighbouring fibrils become too weak to be detected by the imaging method in use, and as such we have to calculate the correlation length from measurements of nearest-neighbour registry and our statistical model. We perform the mapping of the registry data to the strain data by plotting equation (2) using the experimental values for the registry order parameter, S , measured at the various values of the rigidity, E . The only adjustable factor is the strength of the force dipole density of the sarcomere ρ *. The value of E * is given by the peak of the registry data. The mapping is illustrated in Fig. 3 and shows the connection between the structure (registry) and function (strain), which is the central result of this paper. The theoretically predicted strain on the basis of the mapping from zbb measurements are found to match closely with the measured strain values up to a normalization factor corresponding to the magnitude of a cardiomyocyte sarcomere’s contractile forces. Considering about 100 myosin filament heads in a sarcomere, each producing a contractile force of about 1 pN, a reasonable estimate for the contractile force per sarcomere [19] would be ρ *=100 pN, and for typical choices a ~1 μm and E *~5 kPa, we estimate strain magnitudes of about 5 %, quite close to the strains observed in experiment. This connection between strain and registry, two essentially distinct measurements, as depicted graphically in Fig. 3 , is the central result of this paper. 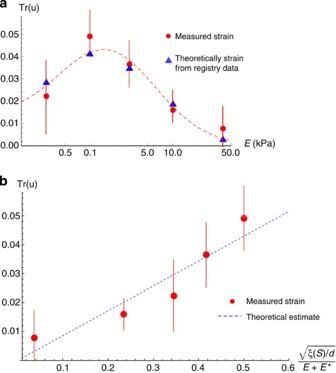Figure 3: Theory matches measured registry order and strain. (a) The z-band breadth data (zbb) are mapped to strain values using our theoretically derived expressions. The measured strain is shown as solid, red dots together with the experimental error bars. The dashed red line is an interpolated guide to the eye that joins the measured strain data points within their error bars. The blue triangles represent the strain values obtained by the theoretical mapping from the corresponding zbb measurements (for the same values of substrate elasticity) and show a close match with the experimentally measured strain values within the error bars. (b) The measured strain is plotted against the corresponding value of the expression, given in equation (2), which is the central result of this paper. The dashed line shows a theoretically estimated straight line (using typical values for force dipole densityρ*=100 pN, and for sarcomere lengtha=1.2 μm), whereas the measured values of the trace of strain are shown as solid red dots. Thus, to within the experimental error, and within some uncertainty of estimating the contractile forces, the data match our theory. Figure 3: Theory matches measured registry order and strain. ( a ) The z-band breadth data (zbb) are mapped to strain values using our theoretically derived expressions. The measured strain is shown as solid, red dots together with the experimental error bars. The dashed red line is an interpolated guide to the eye that joins the measured strain data points within their error bars. The blue triangles represent the strain values obtained by the theoretical mapping from the corresponding zbb measurements (for the same values of substrate elasticity) and show a close match with the experimentally measured strain values within the error bars. ( b ) The measured strain is plotted against the corresponding value of the expression , given in equation (2), which is the central result of this paper. The dashed line shows a theoretically estimated straight line (using typical values for force dipole density ρ *=100 pN, and for sarcomere length a =1.2 μm), whereas the measured values of the trace of strain are shown as solid red dots. Thus, to within the experimental error, and within some uncertainty of estimating the contractile forces, the data match our theory. Full size image Qualitative trends in registry peak as a function of noise Although the mapping in Fig. 3 is our main result, we can also qualitatively analyse the difference in zbb peaks’ height and width between myofibrils and premyofibrils as described by Majkut et al . [8] This difference in the extent of ordering and in peak width of registry order versus substrate elasticity, as shown in Fig. 4b , can be interpreted to be a result of the differences in strength of elastic interaction relative to noise. 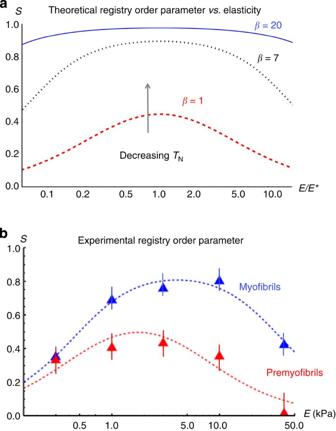Figure 4: Theoretical and experimental dependence of myofibril registry on substrate stiffness. (a) Nearest-neighbour registry correlations, a theoretical measure of the registry of adjacent muscle fibres, as a function of the substrate elasticity at three different values of noise parametrized byβ=Uint/(kBTN), whereTNis an effective temperature. The fibres have the maximum tendency to align at the optimal substrate rigidityE=E*. At lower effective temperatures (higher values ofβ), the muscle fibres show a higher degree of registry over a larger range of substrate elasticities, thus givingbroader as well as higherpeaks. These plots just show qualitative trends and are not meant to be fits to the experimental data. (b) Experimental registry order parameter from z-band breadth measurements: replotted data with permission from Majkutet al.8The z-band breadth is a measure of the nearest-neighbour correlations between fibrils. We define an order parameterSthat varies between 0 and 1 based on such nearest-neighbour correlations. Myofibrils in culture are seen to be more registered than premyofibrils, having a peakSvalue of about 0.8, whereas the corresponding value for premyofibrils is about 0.35. In addition, the myofibril peak is also broader, being 50 kPa at half maximum, whereas the premyofibril peak is only about 10 kPa wide. These are presumably because the premyofibrils are at an early stage of development and characterized by lower contractile forces and more structural disorder, and therefore higher relative noise (lowβ). The dashed lines serve as interpolated guides to the eye that join the data points to within error margins, and are not fits. Figure 4: Theoretical and experimental dependence of myofibril registry on substrate stiffness. ( a ) Nearest-neighbour registry correlations, a theoretical measure of the registry of adjacent muscle fibres, as a function of the substrate elasticity at three different values of noise parametrized by β = U int /( k B T N ), where T N is an effective temperature. The fibres have the maximum tendency to align at the optimal substrate rigidity E = E *. At lower effective temperatures (higher values of β ), the muscle fibres show a higher degree of registry over a larger range of substrate elasticities, thus giving broader as well as higher peaks. These plots just show qualitative trends and are not meant to be fits to the experimental data. ( b ) Experimental registry order parameter from z-band breadth measurements: replotted data with permission from Majkut et al . [8] The z-band breadth is a measure of the nearest-neighbour correlations between fibrils. We define an order parameter S that varies between 0 and 1 based on such nearest-neighbour correlations. Myofibrils in culture are seen to be more registered than premyofibrils, having a peak S value of about 0.8, whereas the corresponding value for premyofibrils is about 0.35. In addition, the myofibril peak is also broader, being 50 kPa at half maximum, whereas the premyofibril peak is only about 10 kPa wide. These are presumably because the premyofibrils are at an early stage of development and characterized by lower contractile forces and more structural disorder, and therefore higher relative noise (low β ). The dashed lines serve as interpolated guides to the eye that join the data points to within error margins, and are not fits. Full size image The substrate-mediated elastic interaction between two fibrils can be tuned by varying the substrate stiffness, E . Equation (1) shows that the interaction is maximal when E = E *, where E * is the rigidity at which the cell force saturates to its maximal value. The interaction falls off to small values for substrates that are too stiff to deform. It is also small on soft substrates where the cells do not reach their fully contractile state. In the absence of noise, the system is perfectly registered even in the presence of infinitesimally small elastic interactions. On the other hand, registry order can be greatly reduced when the noise is larger than the strength of the elastic forces, which is necessarily the case for large or small enough values of the substrate elasticity, where κ ( E ) is small, as suggested by equation (1). A theoretical expression of the order parameter S ( βκ ) is obtained from a statistical physics consideration of the competition between elastic interaction energy, U int , and noise, T N (see Methods for the derivation of an expression for S ), and shows a peak in amplitude as a function of the substrate rigidity corresponding to the maximal strength of elastic forces. At very small or large values of the substrate rigidity, the noise dominates the elastic, registry-promoting, interactions thus suppressing the registry. The rigidity ranges over which this suppression occurs become wider as the noise increases; thus, the rigidity range over which the system shows registry gets narrower. This is consistent with the experimental observation that premyofibrils in isolated cells in culture exhibit both lower degrees of registry (smaller peak order parameter) and narrower peaks in plots of the registry order versus substrate elasticity [8] , as shown in Fig. 4 . Premyofibrils are subject to greater relative noise than are mature myofibrils because of the lower contractility and the higher degree of noise expected in an earlier stage of development. Figure 4b is based on the data presented in Fig. 4f in ref. 8 . The graph compares the registry data for myofibrils and premyofibrils in culture and also for cardiac muscle tissue. There is insufficient data to draw quantitative conclusions about the registry of cardiac tissue in vivo , which seems to have a narrower peak versus elasticity. Moreover, because of the splaying and overlaying of the myofibrils in tissue we do not expect our model, based on the simplified assumption of parallely oriented fibrils on the surface of a substrate, to be directly applicable to this case. We consider a minimal model for striation based on substrate-mediated, elastic interactions between neighbouring myofibrils. With the assumption that in-phase beating of a heart muscle cell occurs only for registered groups of fibrils, we show how one can map the structural (registry) data onto the cardiomyocyte function (beating strain). Both sets of data are related to the same optimal elasticity E * at which the interactions peak, but the strain data peak is shifted from the registry peak because of an additional factor of 1/( E + E *). This illustrates the predictive power of the theory and suggests further experimental tests of our assumed relation between structural registry and in-phase beating of fibril groups. The relative strength of elastic interactions to inherent noise, expressed as a parameter β , is able to provide us with some insight into the differences in extent of registry between myofibrils and premyofibrils. Previous experiments also show that the peak in striation versus substrate elasticity becomes broader and higher with increased development time [16] , suggesting that the system is dynamically evolving towards a less noisy and more registered configuration (see Supplementary Notes 1 and 2 ). We would need to know microscopic details such as the size and spacing of sarcomeres and the contractile forces generated by them, along with the strength of noise, in order to compare the registry data for myofibrils and premyofibrils in a more quantitative manner. In addition, as mentioned above, the strength of the elastic interactions depends on the spacing between neighbouring fibrils whose average and fluctuations may reflect the extent of nematic (orientational) disorder between neighbouring fibrils. We might expect premyofibrils to show less orienational order and hence a larger range of interfibril spacings, resulting in weaker elastic interactions and larger values of β . However, we show that the zbb data can be mapped to the measured strain using a theoretically calculated expression relating beating strain to the registry order parameter, without any explicit knowledge of the strength of noise or of the details of the nematic disorder. In addition to measuring both registry and the extent of nematic order in the same cells, it would be interesting to measure the kinetics of myofibrils in culture that are initially out of registry. Our model predicts (see Supplementary Note 2 ) that striation order should evolve in time with a rate that depends on the substrate elasticity. Registry should be established most rapidly at the optimal substrate stiffness where the elastic forces driving the fibrils towards registry are the largest. Also, the kinetics of evolution of registry could be markedly slowed down by high activation energy barriers corresponding to internal deformations and re-arrangements of the sarcomeres. This could occur over a few days or weeks, time scales that are relevant in development. Our idealized model considers parallel fibrils directly adhered to the substrate and while some of the orientational disorder can be taken into account by an effective reduction of the interaction strength, it is not directly applicable to real cardiac tissue characterized by branching, splaying and overlaid fibrils in a three-dimensional space. However, we believe that with some generalization, the concepts presented here could also provide insights for understanding qualitative trends in both the registry and beating amplitude of heart tissue. Although myofibrillogenesis in differentiating muscle cells in a developing embryo is probably driven by a host of mechanisms to achieve ordering of the stress fibres and developing myofibrils, mechanical signalling as envisaged in our model may be the cue that initiates the registry process, which is in turn related to the coherent beating of the heart muscle cell. Registry order and correlations in steady state A sarcomere is driven into registry with neighbouring fibrils by elastic forces from the substrate that act on it via the adhesion sites at the z-discs. These elastic forces arise from the substrate deformations induced by the neighbouring contractile fibrils and can be derived from the interaction energy of equation 1, which suggests that the forces are zero only if the sarcomere is perfectly registered. In other words, if the sarcomere is registry mismatched with a non-zero phase Δ θ =2 π Δ x / a as defined in the main text, it is acted upon by a force that drives it towards registry, that is, in a direction that tends to reduce Δ x . The sarcomere adhesions are also acted upon by active stochastic forces that cause them to randomly probe these different directions. Such noise can arise from both the contractile action of myosin motors as well as the polymerization of actin filaments. The net elastic force on an adhesion can be represented as the total interaction energy for an assembly of N , such as parallel fibrils, written here as the sum of work done when the adhesion of the sarcomeres is moved in the strain field of its two nearest-neighbouring fibrils (since it can be shown [19] that the strain field induced by a fibril decays exponentially in the transverse y -direction) as, where θ i , j represents the registry mismatch between the j th fibril and the corresponding sarcomere on the i th fibril (see Supplementary Fig. 1 ), and U 0 is the substrate-dependent strength of interaction. This is just a sum of interaction energies defined in equation 1 in the main text. As this equation shows, this is identical to a model of two-dimensional (2D) planar rotors (commonly known as ‘XY model’) [30] , where each rotor or spin vector σ i is described by just one phase angle as it is free to rotate in the 2D plane, , and the interaction energy of any such pair of rotors is proportional to the cosine of the angle between them (as is expected for exchange coupling between spins on a lattice in a model magnetic system). Furthermore, the planar rotor model with nearest-neighbour interactions on a one-dimensional lattice is exactly solvable [30] . In particular, we are interested in a measure of the extent of the striation and of the registry correlations of adjacent (but not necessarily nearest-neighbour) fibrils. This (transverse) correlation length signifies the degree to which fibrils within that distance are registered, which we assume determines the beating strain as explained in the main text. The experimentally measured zbb considers only how closely the Z-bodies of an ensemble of individual sarcomeres in two nearest-neighbour fibrils line up, and as such is related to the nearest-neighbour correlation function of two planar rotors, S . This is a statistically averaged quantity that reflects the noise present in the system, which tends to counteract perfect registry. The nearest-neighbour correlation function can be exactly evaluated as, where the registry mismatch is defined as a phase Δ θ ≡2 π Δ x / a , β = U int /( k B T N ) is the effective noise parameter defined earlier, κ =4 η /(1+ η ) 2 is a peaked function of the non-dimensionalized elasticity η = E / E *, and S ( x )= I 1 ( x )/ I 0 ( x ) is the ratio of modified Bessel functions (of the first kind). The integrals in equation (4) are just the equilibrium statistical average of the order parameter with the interaction energy of equation (1), which enters a Boltzmann factor where the noise [31] is modelled by an effective temperature. To calculate the correlation length that is a measure of the number of fibres whose sarcomeres are in registry, we ask how rapidly the registry correlation of sarcomeres decays as a function of their transverse separation. Consider for example, the correlation of two fibrils, g ( y ), that are separated by y lattice sites in one-dimension. For interactions limited to nearest neighbours, the correlation function between two distant sarcomeres can be written as a product of the nearest-neighbour correlation functions as [30] , The definition of the correlation length ξ (in units of the ‘lattice spacing’, that is, the transverse separation between neighbouring fibrils, d ) follows from the nearest-neighbour correlation function S defined in equation (4) as Physically, this just says that the registry correlations of a given sarcomere with another that is a transverse distance y (in units of the lattice periodicity) away is just given by the product of the central sarcomere with its nearest neighbour and that neighbour with its nearest neighbour 2 lattice sites away, and so on. The correlation length diverges for small noise (relative to the elastic interactions) as ξ ~ κβ (defined above where β is the ratio of the interaction strength and the noise modelled as an effective temperature. The correlation length goes to zero logarithmically for very high effective temperatures, as ξ ~− d /log( βκ ). The correlation length increases monotonically as a function of β , which is expected since the sarcomere registry is more correlated when the elastic interactions dominate the noise. The correlation length diverges for small effective temperatures (relative to the elastic interactions) as ξ ~1/ T N , and goes to zero logarithmically for very high temperatures, as ξ ~ d /log( T N ). Registry-based model for strain We assume that fibrils that lie within a distance ξ of each other constitute a group that beats in phase. Supposing that there are a total of n fibrils within a cell, each separated from its neighbours by a distance d ; it follows then that they can be divided into N = nd / ξ = L / ξ coherently beating groups, L being a length-scale characteristic of the lateral cell size, such that within a group the fibrils beat in phase while we assume that the N groups each beat with a characteristic temporal phase θ i , which is random and uncorrelated with the phase of beating of other groups of fibrils as schematically illustrated in Supplementary Fig. 2 . The measured average substrate strain during a beat (minus the strain during the non-beating time) is the average of the individual strains generated by the contractile fibrils at several points in the substrate around the edge of the cell. The strain produced by each fibril, an array of contractile force dipoles, decays exponentially with distance away from the fibril [19] , and as such the strain at a particular point of the substrate close to the edge of the cell is to a good approximation generated by the nearest myofibril. The strain averaged over all n fibrils is then given by, where ρ ( E ) is the force dipole density that saturates with substrate elasticity as ρ ( E )= ρ */(1+ E / E *), a is the sarcomere length and ω is the frequency of beating. As fibrils within the same correlated group beat with the same phase, the sum over phases in the above equation can be grouped as . The experimentally measured beating strain is an averaged quantity both spatially over the different points of measurement, as well as over the period of a beat. The root mean square of the phase factors averaged over the period of a beat results in an effective prefactor A , that goes as because the phases of the N different groups of fibrils are totally uncorrelated. Here, the ‹ › indicates time averaging over a period of beating. Using the factor of A from equation (8) to represent the time average over the phases in the expression for spatially averaged strain in equation (7), we obtain a theoretical expression for the experimentally measured value of substrate strain at the edge of the cell, where the scaling with substrate elasticity E as a factor of 1/( E + E *) (that is responsible for shifting the strain peak relative to that of registry) and with the correlation length as are the key to understanding the mapping of the registry to strain as discussed in the main body of the paper. This is in the spirit of an approximate scaling relation and the exact magnitude of the strain will depend on microscopic quantities such as the contractile force generated by the myosin motors for each myofibril, which can be reasonably estimated but not exactly calculated. How to cite this article : Dasbiswas, K. et al . Substrate stiffness-modulated registry phase correlations in cardiomyocytes map structural order to coherent beating. Nat. Commun. 6:6085 doi: 10.1038/ncomms7085 (2015).